hVps41 and VAMP7 function in direct TGN to late endosome transport of lysosomal membrane proteins Targeted delivery of lysosome-associated membrane proteins is important for lysosome stability and function. Here we identify a pathway for transport of lysosome-associated membrane proteins directly from the trans- Golgi network to late endosomes, which exists in parallel to mannose 6-phosphate receptor and clathrin-dependent transport of lysosomal enzymes to early endosomes. By immunoelectron microscopy we localized endogenous LAMP-1 and -2 as well as LAMP-1-mGFP to non-coated, biosynthetic carriers at the trans -Golgi network and near late endosomes. These LAMP carriers were negative for mannose 6-phosphate receptor, adaptor-protein complex-1, secretory albumin and endocytic markers, but contained the homotypic fusion and protein sorting complex component hVps41 and the soluble N -ethylmaleimide-sensitive factor attachment protein receptors protein VAMP7. Knockdown of hVps41 or VAMP7 resulted in the accumulation of lysosome-associated membrane protein carriers, whereas knockdown of hVps39 or hVps18 did not, indicating that the effect of hVps41 is independent of CORVET/HOPS. Mannose 6-phosphate receptor carriers remained unaffected upon hVps41 or VAMP7 knockdown, implicating that hVps41 and VAMP7 are specifically involved in the fusion of trans -Golgi network-derived lysosome-associated membrane protein carriers with late endosomes. Lysosomes are the primary catabolic compartments of eukaryotic cells [1] . A functional lysosome requires two classes of proteins: soluble lysosomal acid hydrolases and integral lysosomal membrane proteins. The approximately 25 known lysosomal membrane proteins [2] have diverse functions, including acidification of the lysosomal lumen, protein import and export from and to the cytosol [3] , homo- and heterotypic lysosomal fusion and maintaining integrity of the lysosomal membrane [3] . Newly synthesized lysosomal proteins can take a direct trans-Golgi network (TGN)-to-endosome pathway or an indirect pathway, involving transport to the plasma membrane and subsequent endocytosis. The best understood direct TGN-to-endosome pathway is mannose 6-phosphate receptor (MPR)-dependent transport of lysosomal hydrolases. MPRs bind to the heterotetrameric adaptor-protein complex (AP)-1 and the Golgi-localized, γ-ear-containing, Arf-binding family of proteins (GGA) that both act as clathrin adaptors [4] , [5] . Subsequent transport to endosomes occurs via 60–100 nm clathrin-coated vesicles [5] , [6] , [7] or pleiomorphic membranes [8] that fuse with early endosomes [7] , [9] . Considerably less is known about the targeting of lysosomal membrane proteins [10] . The lysosome-associated membrane proteins (LAMP)-1 and -2 are the most abundant lysosomal membrane proteins [11] . They bear a GYXXØ sorting motif in their cytosolic tail that interacts with the μ subunits of AP-1, AP-2 and AP-3, which are adaptor-protein complexes implicated in vesicle formation at the TGN/endosome, plasma membrane and recycling endosomes, respectively [12] . In accordance, LAMP-1 has been found in AP-1/clathrin positive TGN-derived vesicles [13] , [14] . Several observations, however, indicate that in the absence of AP-1 and/or clathrin or when the GYXXØ motif is mutated, LAMPs still reach lysosomes by a direct pathway [15] , [16] , [17] , [18] . The characteristics of this alternative pathway have thus far remained unresolved. Here, we provide evidence that LAMPs, but not MPRs, can be exported from the TGN via non-clathrin-coated carriers that travel directly to late endosomes. These carriers contain hVps41 as well as the soluble N -ethylmaleimide-sensitive factor attachment protein receptors (SNARE) protein VAMP7, which are both required for fusion with endosomes. The TGN distribution of LAMP-1 and -2 differs from CI-MPR At steady state, the majority of LAMP-1 and LAMP-2 resides in late endosomes and lysosomes with only low levels in the TGN. As a consequence, the localization of LAMPs to distinct TGN subdomains has remained enigmatic. Here, by using an optimized immunoEM protocol [19] , we succeeded to visualize endogenous LAMPs in the TGN with sufficient sensitivity to quantitatively study their distribution in direct comparison with other proteins ( Fig. 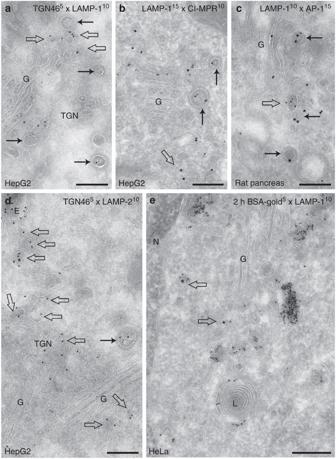Figure 1: LAMP-1 and LAMP-2 distribute differentially over TGN membranes compared to the CI-MPR. Electron micrographs of ultrathin cryosections showing the TGN distributions of endogenous LAMP-1 and LAMP-2 in HepG2, rat pancreatic beta cells and HeLa cells. (a) LAMP-1 (10 nm gold) is present in small vesicles that lack a clathrin coat; the LAMP carriers (open arrows). Closed arrows point to clathrin-coated vesicles, which can also contain LAMP-1. (b) LAMP-1-positive (15 nm gold) LAMP carriers (open arrows) are negative for CI-MPR (10 nm gold) and can display an internal membrane (asterisk; *). CI-MPR is found in clathrin-coated vesicles (closed arrows). (c) LAMP carriers (open arrow) are positive for LAMP-1 (10 nm gold), but devoid of AP-1 label (15 nm). Closed arrows point to AP-1/clathrin-coated vesicles. (d) LAMP-2 (10 nm gold) is also found in LAMP carriers (open arrows). TGN46 (5 nm gold particles) is a marker for TGN membranes. (e) LAMP carriers (labelled by LAMP-1, 10 nm gold) in HeLa cells pre-loaded with BSA-gold5for 2 h. E, endosome; G, Golgi; L, Lysosome; N, Nucleus; TGN,transGolgi network. The asterisks (*) in LAMP carriers indicate the presence of an internal membrane. Scale bar, 200 nm. 1 , Table 1 and Supplementary Fig. S1 ). Figure 1: LAMP-1 and LAMP-2 distribute differentially over TGN membranes compared to the CI-MPR. Electron micrographs of ultrathin cryosections showing the TGN distributions of endogenous LAMP-1 and LAMP-2 in HepG2, rat pancreatic beta cells and HeLa cells. ( a ) LAMP-1 (10 nm gold) is present in small vesicles that lack a clathrin coat; the LAMP carriers (open arrows). Closed arrows point to clathrin-coated vesicles, which can also contain LAMP-1. ( b ) LAMP-1-positive (15 nm gold) LAMP carriers (open arrows) are negative for CI-MPR (10 nm gold) and can display an internal membrane (asterisk; *). CI-MPR is found in clathrin-coated vesicles (closed arrows). ( c ) LAMP carriers (open arrow) are positive for LAMP-1 (10 nm gold), but devoid of AP-1 label (15 nm). Closed arrows point to AP-1/clathrin-coated vesicles. ( d ) LAMP-2 (10 nm gold) is also found in LAMP carriers (open arrows). TGN46 (5 nm gold particles) is a marker for TGN membranes. ( e ) LAMP carriers (labelled by LAMP-1, 10 nm gold) in HeLa cells pre-loaded with BSA-gold 5 for 2 h. E, endosome; G, Golgi; L, Lysosome; N, Nucleus; TGN, trans Golgi network. The asterisks (*) in LAMP carriers indicate the presence of an internal membrane. Scale bar, 200 nm. Full size image Table 1 Concentration of LAMPs and CI-MPR in clathrin-coated TGN membranes. Full size table In both HepG2 ( Fig. 1a ) and rat pancreatic beta cells ( Supplementary Fig. S1a ) LAMP-1 label could be detected in the trans -Golgi/TGN cisterna that also contained the TGN markers TGN46 ( Fig. 1a ) or TGN38 ( Supplementary Fig. S1a ). In the reticulated TGN membranes, LAMP-1 was predominantly found in non-coated, 70–200 nm diameter vesiculo-tubular membranes that we designated ‘LAMP carriers’ (open arrows in Fig. 1a and Supplementary Fig. S1a ). In addition, some LAMP-1 was seen in clathrin-coated membranes (arrows in Fig. 1a and Supplementary Fig. S1a ) [13] . Notably, LAMP carriers lacked a clathrin coat and were devoid of label for cation-independent (CI)-MPR ( Fig. 1b ) and AP-1 ( Fig. 1c ). CI-MPR—as expected—was readily found in clathrin-coated membranes ( Fig. 1b , refs 7 , 20 , 21 and Supplementary Fig. S1b,c ), in which its labelling density was 2.8 × concentrated over non-coated TGN membranes ( Table 1 ). LAMP-1 was not concentrated in coated TGN membranes ( Table 1 ). A similar localization was observed for LAMP-2 ( Fig. 1d ). LAMP-2 was also found in LAMP carriers and only moderately enriched in clathrin-coated TGN membranes ( Table 1 ). These data indicate that LAMPs can enter a specialized TGN domain, the LAMP carriers, as well as clathrin-coated TGN membranes. In the clathrin-coated TGN membranes, however, LAMPs are not concentrated, or less concentrated than CI-MPR. LAMP carriers were also found at distance from the TGN, that is, dispersed in the cytosol, near endosomes ( Figs 1d and 2b–e ) and at the cell periphery (not shown). Typically, they regularly contained an internal membrane (asterisks in Fig. 1b ). Similar carriers were observed in various cell types, including HeLa ( Fig. 1e ), NRK, MDCK and fibroblasts (not shown). The number of LAMP carriers per cell profile was relatively low. Ultrathin sections of HepG2 cells contained ~3–4 LAMP carriers per cell profile (LAMP-1 labelling: 131 carriers in 44 cell profiles; LAMP-2 labelling: 148 in 34 cell profiles), although some cells displayed local accumulations around late endosomes ( Fig. 2b ). In HeLa cells on average 2 LAMP carriers were present per cell profile. 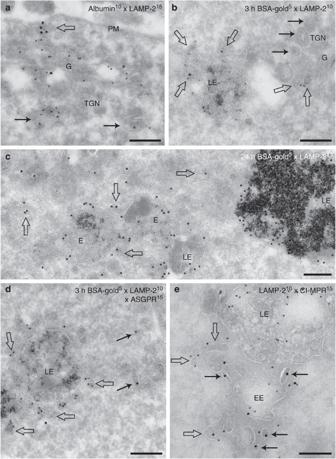Figure 2: Characterization of TGN and late endosome-associated LAMP carriers. Electron micrographs of ultrathin cryosections of HepG2 cells showing LAMP carriers in the TGN and in close association with late endosomes. Cells shown in (b,d) were incubated 3 h with BSA-gold5before fixation and in (c) 24 h with BSA-gold5before fixation. (a) A LAMP carrier (open arrow) positive for LAMP-2 (15 nm gold) is negative for the secretory protein albumin (10 nm gold). Albumin is found in constitutive secretory vesicles (closed arrows), which are morphologically distinct from LAMP carriers. (b) LAMP-2 (10 nm gold)-positive LAMP carriers (open arrows) are found in the TGN and near late endosomes (LE). Closed arrows indicate TGN-associated clathrin-coated vesicles. The LE contains endocytosed BSA-gold5, which is absent from the LAMP carriers. (c) LAMP-2 (10 nm gold)-positive LAMP carriers (open arrows) in close association with LE. Despite abundant labelling of the endosomes (E) with internalized BSA-gold5(24 h uptake) the LAMP carriers are negative for this endocytic marker. (d) LAMP-2 (10 nm gold)-positive LAMP carriers (open arrows) are distinct from ASGPR (15 nm gold)-containing recycling vesicles (arrows). (e) LAMP-2 (10 nm gold)-positive LAMP carriers near E (open arrows) are different from CI-MPR (15 nm gold)-containing carriers (arrows). EE, Early endosome; E, Endosome; G, Golgi; LE, late endosome; PM, plasma membrane; TGN,transGolgi network. Scale bar, 200 nm. Figure 2: Characterization of TGN and late endosome-associated LAMP carriers. Electron micrographs of ultrathin cryosections of HepG2 cells showing LAMP carriers in the TGN and in close association with late endosomes. Cells shown in ( b , d ) were incubated 3 h with BSA-gold 5 before fixation and in ( c ) 24 h with BSA-gold 5 before fixation. ( a ) A LAMP carrier (open arrow) positive for LAMP-2 (15 nm gold) is negative for the secretory protein albumin (10 nm gold). Albumin is found in constitutive secretory vesicles (closed arrows), which are morphologically distinct from LAMP carriers. ( b ) LAMP-2 (10 nm gold)-positive LAMP carriers (open arrows) are found in the TGN and near late endosomes (LE). Closed arrows indicate TGN-associated clathrin-coated vesicles. The LE contains endocytosed BSA-gold 5 , which is absent from the LAMP carriers. ( c ) LAMP-2 (10 nm gold)-positive LAMP carriers (open arrows) in close association with LE. Despite abundant labelling of the endosomes (E) with internalized BSA-gold 5 (24 h uptake) the LAMP carriers are negative for this endocytic marker. ( d ) LAMP-2 (10 nm gold)-positive LAMP carriers (open arrows) are distinct from ASGPR (15 nm gold)-containing recycling vesicles (arrows). ( e ) LAMP-2 (10 nm gold)-positive LAMP carriers near E (open arrows) are different from CI-MPR (15 nm gold)-containing carriers (arrows). EE, Early endosome; E, Endosome; G, Golgi; LE, late endosome; PM, plasma membrane; TGN, trans Golgi network. Scale bar, 200 nm. Full size image LAMP carriers are not constitutive secretory vesicles A major TGN-derived pathway is clathrin-independent transport to the plasma membrane [22] . As LAMPs can follow this pathway as part of the indirect pathway to lysosomes, we investigated whether LAMP carriers represent constitutive secretory vesicles. Double-immunogold labelling for LAMP-1 and albumin, a constitutive secretory protein of HepG2 cells, visualized albumin in the Golgi complex, in non-coated vesicles in the TGN area and en route to the plasma membrane ( Fig. 2a ). These albumin-positive vesicles were distinct from LAMP carriers by their irregular shape, dense content and lack of internal membranes [23] ( Fig. 2a ). Moreover, quantitative analysis showed that 37% of the labelled TGN vesicles contained only LAMP-1, 61% only albumin, whereas only 2% contained both proteins. These data show that LAMP carriers differ from constitutive secretory vesicles en route to the plasma membrane. TGN-derived LAMP carriers concentrate around late endosomes We regularly observed LAMP carriers near endosomes (for example, Fig. 2b–e ). This was confirmed by quantitative analysis, revealing that within the plane of an ultrathin section >40% of the LAMP carriers is found in close association (that is, within a distance of 150 nm) of endosomes. Of these endosome-associated LAMP carriers 58% of the LAMP-1 and 67% of the LAMP-2-positive carriers were associated with late endosomes, that is, containing more than 8 intraluminal vesicles [20] . Notably, LAMP-1 or -2-positive carriers were consistently negative for BSA-gold 5 , also when HepG2 cells were incubated for 24 h with BSA-gold 5 or when they surrounded endosomes with high concentrations of BSA-gold 5 ( Fig. 2c ). The association of LAMP carriers with late endosomes differs from the distribution of AP-3 and SNX1-positive carrier vesicles [20] , [21] , which mediate exit of lysosomal membrane proteins and MPRs, respectively, from early endosomal intermediates. In agreement herewith, LAMPs and CI-MPR resided in different subpopulations of endosome-associated vesicles ( Fig. 2e ) [5] , [6] , [7] . LAMP carriers also lacked asialoglycoprotein receptor (ASGPR) ( Fig. 2d ), a marker for recycling endosomes. Together these data show that LAMP carriers away from the TGN lack endocytic cargo, CI-MPR and ASGPR and are often found in close association with late endosomes, suggesting that they transport LAMPs from the TGN to late endosomes. LAMP-1-mGFP carriers travel from TGN to late endosomes To further study the directionality of LAMP carrier transport, we transfected cells with LAMP-1-mGFP and prepared ultrathin cryosections immunogold labelled for green fluorescent protein (GFP) in order to detect newly synthesized LAMP-1 only. Sixteen hours after transfection we found LAMP-1-mGFP in LAMP carriers surrounding late endosomes with no or very low detectable levels of LAMP-1-mGFP ( Fig. 3a ). In other cells we could find LAMP-1-mGFP label at the limiting membrane of late endosomes/lysosomes, illustrating that the construct is correctly targeted ( Fig. 3b ; for fluorescent staining pattern see Supplementary Fig. S2 ). To increase LAMP-1-mGFP labelling in the Golgi/TGN we applied a 20°C block, which delays TGN exit [24] . Cells were fixed 15–20 min after release of the block. This resulted in elevated levels of LAMP-1-mGFP in the Golgi cisternae and TGN and the occurrence of numerous LAMP-1-mGFP-positive LAMP carriers ( Fig. 3c ). Notably, we regularly found LAMP-1-mGFP-positive carriers in close proximity to endosomes that had not yet received detectable levels of newly synthesized LAMP-1-mGFP ( Fig. 3d ), which is consistent with the scenario that LAMP carriers mediate direct transport of LAMPs from the TGN to late endosomes. 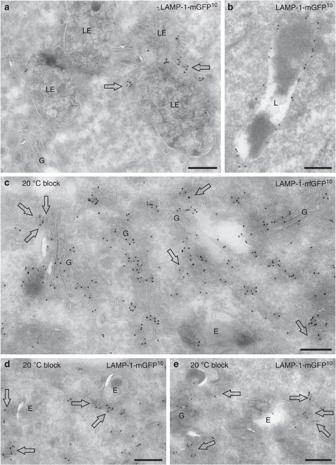Figure 3: LAMP carriers contain newly synthesized LAMP-1-mGFP. Electron micrographs of ultrathin cryosections of HepG2 cells 7 h after transfection with LAMP-1-mGFP and labelled with anti-GFP (10 nm gold) to detect newly synthesized LAMP-1-mGFP. In (c–e) a 20-°C TGN exit block was induced for 1 h. Cells were fixed 10–15 min after release of the temperature block. (a) LAMP carriers (open arrows) containing LAMP-1-GFP are closely associated with late endosomes (LE) with no or low labelling levels, in accordance with the proposed role for LAMP carriers in delivering LAMPs to LE. (b) The LAMP-1-mGFP construct is properly targeted to lysosomes (L). (c) A 20-°C TGN block gives rise to numerous LAMP carriers in the TGN area. (d) Block of 20 °C. LAMP-1-mGFP-positive LAMP carriers (open arrows) are found close to unlabeled endosomes (E). (e) Block of 20 °C. A LAMP-1-mGFP-positive Golgi complex and several labelled LAMP carriers (open arrows) are seen in close proximity to unlabeled endosomes (E). E, Endosome; G, Golgi; LE, Late endosome; L, Lysosome. Scale bar, 200 nm. Figure 3: LAMP carriers contain newly synthesized LAMP-1-mGFP. Electron micrographs of ultrathin cryosections of HepG2 cells 7 h after transfection with LAMP-1-mGFP and labelled with anti-GFP (10 nm gold) to detect newly synthesized LAMP-1-mGFP. In ( c – e ) a 20-°C TGN exit block was induced for 1 h. Cells were fixed 10–15 min after release of the temperature block. ( a ) LAMP carriers (open arrows) containing LAMP-1-GFP are closely associated with late endosomes (LE) with no or low labelling levels, in accordance with the proposed role for LAMP carriers in delivering LAMPs to LE. ( b ) The LAMP-1-mGFP construct is properly targeted to lysosomes (L). ( c ) A 20-°C TGN block gives rise to numerous LAMP carriers in the TGN area. ( d ) Block of 20 °C. LAMP-1-mGFP-positive LAMP carriers (open arrows) are found close to unlabeled endosomes (E). ( e ) Block of 20 °C. A LAMP-1-mGFP-positive Golgi complex and several labelled LAMP carriers (open arrows) are seen in close proximity to unlabeled endosomes (E). E, Endosome; G, Golgi; LE, Late endosome; L, Lysosome. Scale bar, 200 nm. Full size image To visualize LAMP transport to late endosomes in living cells we transfected HepG2 cells with LAMP-1-mGFP ( Supplementary Fig. S2 ) and labelled the endo–lysosomal system with dextran-Alexa568 (2 h uptake). As LAMPs are enriched in the limiting membrane of late endosomes/lysosomes, LAMP-1-mGFP-positive late endosomes/lysosomes appear as fluorescent ‘rings’ enclosing a core of dextran-Alexa568 ( Supplementary Fig. S2c ). Correlative live-cell imaging–immunoEM confirmed that these ‘ring’ endosomes are indeed late endosomes (see Fig. 2 in [25] ) and Supplementary Fig. S2d . The Golgi region was identified by its elongated compact shape, its position close to the nucleus, the presence of LAMP-GFP after a 20-°C block and the absence of endocytosed dextran ( Supplementary Fig. S2b ). This definition was confirmed by localization of TGN46 when cells were fixed and immuno-labelled after imaging ( Supplementary Fig. S2a ). Importantly, in live cells we found LAMP-1-mGFP-positive spots exiting the Golgi/TGN area and fusing with LAMP-1-mGFP/dextran-Alexa568-positive ‘ring’ endosomes ( Supplementary Fig. S2b and Supplementary Movie 1 ). Although this approach can not reveal the nature of the carriers, it does illustrate that direct Golgi/TGN to late endosome transport of LAMPs occurs in living cells. LAMP carriers contain hVps41 and VAMP7 In yeast, the vacuolar homotypic fusion and protein sorting (HOPS) complex together with the endosomal class-C core vacuole/endosome tethering (CORVET) complex [26] is involved in all endosome-vacuole-associated fusion events [27] . The HOPS complex consists of four cytosolic class-C vacuolar protein sorting (Vps) proteins (Vps11, Vps16, Vps18 and Vps33 (ref. 28 )), which is the class-C core complex that is shared with the CORVET complex. The accessory subunits Vps39 and Vps41 are specific for the HOPS complex [26] . Recently, we found that depletion of hVps41 or its Drosophila homologue ‘Light’ (lt), reduced the co-localization between LAMP-1-GFP and internalized dextran-Alexa in HeLa and Drosophila S2 cells, respectively [29] . This prompted us to explore a possible role for hVps41 in the LAMP carrier pathway. We first established the subcellular localization of hVps41 by expressing HA-tagged hVps41 in HeLa cells. By immunoEM, hVps41-HA localized to the limiting membrane of late endosomes and lysosomes ( Fig. 4a ), which is in agreement with the vacuolar localization of Vps41p in yeast [30] . In addition, hVps41 was found on vesicles with a similar morphology as LAMP carriers. To establish the nature of these vesicles we performed double-immunogold labelling of LAMP-1 and hVps41-HA, which revealed a striking co-localization on the LAMP carriers ( Fig. 4b ). hVps41-HA was also found in the TGN, where it, like LAMPs, showed a markedly distinct distribution than CI-MPR ( Fig. 4c ). These data show that hVps41 is recruited to late endosomes, lysosomes and, unexpectedly, also LAMP carriers. 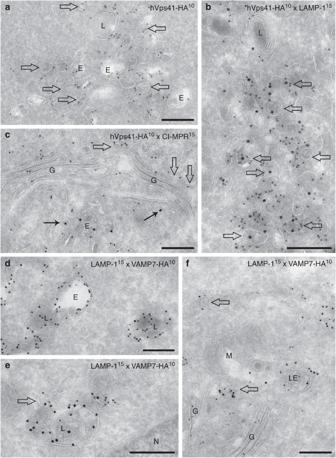Figure 4: hVps41-HA and VAMP7-HA localization. Electron micrographs of ultrathin cryosections of HeLa cells transfected with hVps41-HA or VAMP7-HA and labelled for HA (10 nm gold). (a) hVps41-HA is found on the limiting membrane of endosomes (E) and lysosomes (L), as well as on small vesicles (open arrows). (b) Double labelling for hVps41-HA and LAMP-1 (15 nm gold) showing co-localization on LAMP carriers (open arrows). (c) Double labelling for hVps41-HA and CI-MPR (15 nm gold) reveals distinct localization patterns in the TGN. Open arrows point to hVps41-HA-positive vesicles, closed arrows point to CI-MPR vesicles. (d) VAMP7-HA and LAMP-1 (15 nm gold) co-localize on endosomes (E) and lysosomes (L). (e) VAMP7-HA and LAMP-1 (15 nm gold) co-localize in LAMP carriers (open arrows) closely associated with a lysosome (L). (f) TGN area showing co-localization of VAMP7-HA and LAMP-1 (15 nm gold) on LAMP carriers (open arrows) and a late endosome (LE). E, Endosome; G, Golgi; LE, Late endosome; L, Lysosome; M, Mitochondrion. Scale bar, 200 nm. Figure 4: hVps41-HA and VAMP7-HA localization. Electron micrographs of ultrathin cryosections of HeLa cells transfected with hVps41-HA or VAMP7-HA and labelled for HA (10 nm gold). ( a ) hVps41-HA is found on the limiting membrane of endosomes (E) and lysosomes (L), as well as on small vesicles (open arrows). ( b ) Double labelling for hVps41-HA and LAMP-1 (15 nm gold) showing co-localization on LAMP carriers (open arrows). ( c ) Double labelling for hVps41-HA and CI-MPR (15 nm gold) reveals distinct localization patterns in the TGN. Open arrows point to hVps41-HA-positive vesicles, closed arrows point to CI-MPR vesicles. ( d ) VAMP7-HA and LAMP-1 (15 nm gold) co-localize on endosomes (E) and lysosomes (L). ( e ) VAMP7-HA and LAMP-1 (15 nm gold) co-localize in LAMP carriers (open arrows) closely associated with a lysosome (L). ( f ) TGN area showing co-localization of VAMP7-HA and LAMP-1 (15 nm gold) on LAMP carriers (open arrows) and a late endosome (LE). E, Endosome; G, Golgi; LE, Late endosome; L, Lysosome; M, Mitochondrion. Scale bar, 200 nm. Full size image HOPS/CORVET components interact with Rab-GTPases (Rab7, Rab5 and Rab11) to establish an initial connection between vesicles and their target membrane [31] , [32] , [33] . Subsequent membrane fusion requires pairing of SNAREs. SNARE proteins involved in endo-lysosome fusion are vti-1b, syntaxin7, syntaxin8, VAMP7 and VAMP8 [34] . Interestingly, in PC12 cells, VAMP7 was previously localized on late endosomes as well as on vesicles that resemble LAMP carriers [35] , but the latter were not further characterized. We therefore stably transfected HeLa cells with VAMP7-HA. By immunoEM, VAMP7-HA was localized to late endosomes, lysosomes [35] ( Fig. 4d ) and, indeed, LAMP carriers ( Fig. 4e ). Together these data show that LAMP carriers contain both the fusion machinery proteins hVps41 and VAMP7. LAMP carriers accumulate upon hVps41 or VAMP7 knockdown To determine whether hVps41 and VAMP7 are required for LAMP carrier trafficking we depleted cells of these proteins by using small interfering RNAs (siRNAs) ( Supplementary Fig. S3a–d ). Cells were treated with siRNAs for 3 days, after which the percentage of knockdown was assessed by RT–PCR. On average we obtained a 90% knockdown. By immunoEM, we found that hVps41 knockdown resulted in a significant increase in the number of LAMP carriers per cell profile (6.8±0.66 (average±s.e.m.) in the knockdown cells and 2.1±0.25 in the parallel control) ( Fig. 5a–c and f ), whereas the number of CI-MPR carriers remained the same ( Fig. 5f ). A similar phenotype was observed after VAMP7 knockdown: 4.9±0.42 in the knockdown cells and 1.8±0.22 in the parallel control ( Fig. 5d–f ). 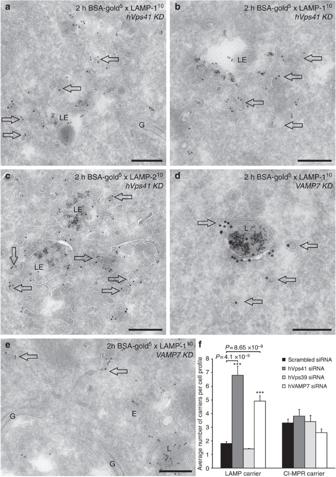Figure 5: hVps41 and VAMP7 knockdown leads to an accumulation of LAMP carriers. Electron micrographs of ultrathin cryosections of HeLa cells treated with hVps41- or VAMP7 siRNAs for 3 days. Cells were incubated with BSA-gold5for 2 h before fixation and immunogold labelled for either endogenous LAMP-1 (a,b,d,e) or LAMP-2 (c). (a) LAMP-1-positive (10 nm gold) LAMP carriers (open arrows) accumulating in hVps41-depleted cells. (b) LAMP-1-positive (10 nm gold) LAMP carriers (open arrows) accumulating around a late endosome (LE) in hVps41 depleted cells. (c) LAMP-2-positive (10 nm gold) LAMP carriers (open arrows) accumulating near BSA-gold5-positive LE in hVps41-depleted cells. (d) LAMP carriers in the proximity of a lysosome (L) in VAMP7 knockdown cells. (e) LAMP carriers in VAMP7 knockdown cells. (f) Quantification of LAMP and CI-MPR carriers in scrambled control, hVps41-, hVps39- or VAMP7 knockdown HeLa cells. Numbers are derived from 40 random cell profiles sampled from at least two EM grids. Control and knockdown cells were treated in parallel, using the same standard buffers. Error bars represent the s.e. of the mean (n=40).P-values were analysed using a two-sidedt-test with unequal variance and related to the scrambled control belonging to that specific experiment (for clarity controls are pooled in the graph). The number of LAMP carriers significantly increases in hVps41- and VAMP7-depleted cells, whereas the number of CI-MPR carriers remains unaffected. E, Endosome; G, Golgi; LE, Late endosome; L, Lysosome. Scale bar, 200 nm. Figure 5: hVps41 and VAMP7 knockdown leads to an accumulation of LAMP carriers. Electron micrographs of ultrathin cryosections of HeLa cells treated with hVps41- or VAMP7 siRNAs for 3 days. Cells were incubated with BSA-gold 5 for 2 h before fixation and immunogold labelled for either endogenous LAMP-1 ( a , b , d , e ) or LAMP-2 ( c ). ( a ) LAMP-1-positive (10 nm gold) LAMP carriers (open arrows) accumulating in hVps41-depleted cells. ( b ) LAMP-1-positive (10 nm gold) LAMP carriers (open arrows) accumulating around a late endosome (LE) in hVps41 depleted cells. ( c ) LAMP-2-positive (10 nm gold) LAMP carriers (open arrows) accumulating near BSA-gold 5 -positive LE in hVps41-depleted cells. ( d ) LAMP carriers in the proximity of a lysosome (L) in VAMP7 knockdown cells. ( e ) LAMP carriers in VAMP7 knockdown cells. ( f ) Quantification of LAMP and CI-MPR carriers in scrambled control, hVps41-, hVps39- or VAMP7 knockdown HeLa cells. Numbers are derived from 40 random cell profiles sampled from at least two EM grids. Control and knockdown cells were treated in parallel, using the same standard buffers. Error bars represent the s.e. of the mean ( n =40). P -values were analysed using a two-sided t -test with unequal variance and related to the scrambled control belonging to that specific experiment (for clarity controls are pooled in the graph). The number of LAMP carriers significantly increases in hVps41- and VAMP7-depleted cells, whereas the number of CI-MPR carriers remains unaffected. E, Endosome; G, Golgi; LE, Late endosome; L, Lysosome. Scale bar, 200 nm. Full size image To test whether the effect of hVps41 knockdown on LAMP carriers was specific for hVps41 or indicative for HOPS complex functioning, we extended our studies to hVps39 (VAM6, TLP). The C-terminal domain of hVps39 shows high homology with the C-terminal domain of yeast Vps39p, the other HOPS-specific component in yeast, which is required for interaction with the class-C core proteins. However, this homology is weak in the N-terminal domain, which contains the Ypt7-/yRab7-binding domain [36] , [37] . Over its entire length, however, hVps39 shows high homology with yeast CORVET component Vps3p, including the N-terminal domain, which binds Vps21p/yRab5 (ref. 36 ). Indeed, hVps39 binds to GST-hRab5 as well as hRab7 (ref. 32 ), both to the GDP and GTP-forms, suggesting that hVps39 could act in the HOPS complex as well as in an intermediate CORVET/HOPS complex, as functional homologue of Vps3p. By immunoEM we localized hVPS39-HA to late endosomes and lysosomes, but LAMP carriers were not significantly labelled [38] . Knockdown of hVps39 did not influence expression levels of hVps41 and vice versa ( Supplementary Fig. S3a,b ). Interestingly, in contrast to hVps41, we found no effect of hVps39 knockdown on the number of LAMP carriers: 1.4±0.01 in the knockdown cells and 1.6±0.03 in the parallel control ( Fig. 5f ). Also the number of MPR carriers remained unaltered in hVps39 knockdown cells ( Fig. 5f ). To extend these data to a core protein of the CORVET/HOPS complex we next induced hVps18 knockdown. Previous studies in various model systems (yeast, D. melanogaster , C. elegans , mice) established a role of Vps18 in lysosome biogenesis [39] , [40] . Three days silencing with siRNA for hVps18 resulted in a 90–96% reduction of hVps18 mRNA and a 22–28% reduction in hVps41 mRNA. The number of LAMP carriers, however, was unaffected: 2.6±0.3 in hVps18 knockdown cells and 2.1±0.2 in the parallel control. These data show that knockdown of VAMP7 and hVps41, but not hVps39 or hVps18, results in the accumulation of LAMP carriers, implying a role for VAMP7 and hVps41 in the fusion of LAMP carriers with endosomes. Over the past decades, numerous observations in the literature have suggested the existence of a clathrin-independent pathway to deliver newly synthesized LAMPs directly from the TGN to the endo–lysosomal pathway [15] , [16] , [17] , [18] . However, the characteristics of this pathway have remained unresolved. Here, we provide the first direct evidence for a clathrin-independent, hVps41 and VAMP7-dependent transport pathway from the TGN to late endosomes that is used by LAMPs, but not MPR. We show that LAMP-1 and -2 in the TGN enter a subpopulation of 70–200 nm diameter vesicles, which lack CI-MPR, clathrin and AP-1, but are positive for hVps41 and VAMP7. We designated these vesicles ‘LAMP carriers’ (characteristics are summarized in Supplementary Fig. S3e ). We propose that LAMP carriers transport LAMPs to late endosomes in a pathway parallel to clathrin-coated carriers [7] , [9] that transport MPRs and lysosomal enzymes to early endosomes. A schematic representation of this model is provided in Fig. 6 . 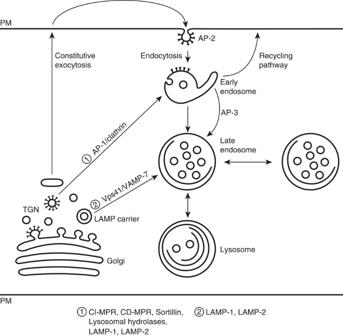Figure 6: Model for differential direct transport pathways of MPR and LAMP carriers. Based on the literature and our present findings we propose that there are at least two main pathways for the direct delivery of newly synthesized lysosomal proteins to the endosomal system: (1) the AP-1/clathrin-mediated pathway to early endosomes (EE) and (2) the LAMP carrier pathways to late endosomes. These pathways differ in cargo, machinery and their site of intersection with endosomes. hVps41 and VAMP7, but not hVps39 or hVps18, are involved in the fusion of LAMP carriers with late endosomes (LE). Figure 6: Model for differential direct transport pathways of MPR and LAMP carriers. Based on the literature and our present findings we propose that there are at least two main pathways for the direct delivery of newly synthesized lysosomal proteins to the endosomal system: (1) the AP-1/clathrin-mediated pathway to early endosomes (EE) and (2) the LAMP carrier pathways to late endosomes. These pathways differ in cargo, machinery and their site of intersection with endosomes. hVps41 and VAMP7, but not hVps39 or hVps18, are involved in the fusion of LAMP carriers with late endosomes (LE). Full size image Our data show that the HOPS component hVps41 and the SNARE VAMP7 are required for the fusion of LAMP carriers with late endosomes. By immunoEM we found that hVps41 and VAMP7 localize to the limiting membrane of late endosomes and lysosomes [30] , as well as to LAMP carriers. Moreover, depletion of hVps41 and VAMP7 resulted in an accumulation of LAMP carriers. Interestingly, knockdown of hVps39 or the class-C core complex component hVps18 did not result in the accumulation of LAMP carriers. These data imply a role for hVps41 in the fusion of LAMP carriers with late endosomes independent of hVps39 and hVps18 and possibly also the other components of the HOPS/CORVET complexes. The presence of hVps41 and VAMP7 on biosynthetic membranes, that is, the LAMP carriers, is remarkable, as both hVps41 and VAMP7 are generally considered endosomal proteins. Plausibly, their localization on LAMP carriers is essential to permit fusion of these carriers with late endosomes. VAMP7, also known as Tetanus toxin Insensitive VAMP (TI-VAMP), belongs to the Longin family of v-SNAREs [41] and has been reported to act in various fusion events involving endosomes and lysosomes: endosome–lysosome fusion [34] , [35] , and fusion of (secretory) lysosomes with the plasma membrane. The LAMP carrier pathway could therefore also function in the delivery VAMP7 to the endo–lysosomal system. A specific role for hVps41 in the transport of LAMP carriers, independent of HOPS, is in concurrence with recent studies on other CORVET/HOPS components. For example, Vps33b can interact with the core class-C proteins of the CORVET/HOPS complexes, but is also found in a complex with VIPAR (Vps33b-interacting protein involved in polarity and apical protein restriction) and Rab11a. The Vps33b–VIPAR–Rab11a complex associates with recycling endosomes and functions in the apical delivery of membrane proteins in polarized cells of humans, mice and zebrafish [42] (and unpublished data of the Klumperman and Gissen labs). Moreover, in yeast and Drosophila, mutations in the core class-C proteins give distinct phenotypes, suggesting that individual subunits have distinct activities [29] , [39] . Thus, specific HOPS components might function in multiple complexes, located at distinct membranes and mediating separate pathways. To investigate this for hVps41, we studied in a parallel study [38] the effects of hVps41 or hVps39 knockdown on endosomal maturation. We found that both hVps41 and Vps39 knockdown affect late endosome fusion and impair the delivery of endocytosed cargo to enzymatically active endo–lysosomal compartments. These data are in agreement with the localization of hVps41 and hVps39 on endosomes and lysosomes (this paper) and indicate that hVps41, in addition to a HOPS-independent function in the LAMP carrier pathway, also participates in lysosomal maturation, probably as part of the HOPS complex. Understanding the role of hVps41 in LAMP transport and endosomal maturation is of interest to comprehend its emerging role in pathologies. An RNAi screen in a C. elegans model for Parkinson’s disease implicated Vps41 in the accumulation of misfolded alpha-synuclein protein [43] . Human gastric and colorectal cancers with high microsatellite instability regularly show frameshift mutations in hVPS41 genes [44] and in a majority of primary effusion B-cell lymphoma cell lines the hVPS41 gene is deregulated [45] . Moreover, hVps41 and other components of the HOPS complex were recently shown to be essential for infection of cells with Ebola virus [46] . These studies indicate hVps41 as an important factor in tumour development and human disease. Yeast Vps41p is recruited to membranes of the endosomal system by activated Ypt7, yeast Rab7, and acidic phospholipids [47] . In preliminary immunoEM studies we found that eGFP-Rab7 and mCherry-Rab7 constructs co-localized with LAMPs on LAMP carriers (Klumperman lab, unpublished data). However, knockdown of Rab7 did not block the formation of LAMP carriers, nor did it impair their fusion with late endosomes, which renders the functional implication of this localization unclear. Recently it was shown that recruitment of hVps41 and HOPS to lysosomes can also occur independent of Rab7 by Arl8b [48] , a member of the Arl (Arf-like) family of GTPases. Interestingly, Arl8b directly interacts with Vps41 (ref. 48 ). Further studies are required to clarify a possible role of Rab7 and/or Arl8b in recruitment of hVps41 to LAMP carriers. Yeast Vps41p also binds AP-3, a heterotetrameric adaptor protein involved in the lysosomal delivery of LAMPs, but not MPR and lysosomal enzymes [12] ( Fig. 6 ). Vps41p has therefore been implicated in AP-3 vesicle biogenesis [49] and/or -fusion [33] . However, in mammalian cells AP-3 predominantly localizes to early endosome-associated tubules [21] ( Fig. 6 ), which are distinct from LAMP carriers. This makes it unlikely that hVps41 is involved in the biogenesis of AP-3 vesicles. Alternatively, it was suggested that Vps41p might be required on the vacuole for fusion of incoming AP-3 vesicles [33] . This scenario would be consistent with the localization of hVps41 and AP-3 in mammalian cells, as hVps41 is present on late endosomes and lysosomes, the likely target for AP-3 vesicles ( Fig. 6 ). The number of MPR carriers was not affected by hVps41, hVps39 or VAMP7 knockdown. This observation is in agreement with the targeting of MPR to relatively early endocytic compartments [9] at a stage before hVps41, hVps39 and VAMP7 functioning ( Fig. 6 ). In yeast the targeting of the soluble lysosomal hydrolase carboxypeptidase Y (CPY) and the integral membrane protein alkaline phosphatase (ALP) require distinct pathways and machinery [50] . ALP is transported directly to the vacuole, in an AP-3 dependent pathway, whereas CPY transport is indirect involving passage over an endosomal intermediate. Mutation of Vps39p (Δvam6) or Vps41p (Δvam2) leads to a partial defect in the processing of CPY, but a complete block in the maturation of ALP [30] . In contrast, deletion of Vps3—or the other CORVET component Vps8—impairs transport of CPY but not ALP [51] , [52] . Our present studies show that while both hVps39 and hVps41 are required for lysosomal maturation, only hVps41 in addition is required for the delivery of LAMP carriers to late endosomes. These findings are in line with the proposed functional homology of hVps39 with yeast Vps3p [32] , [36] , suggesting that hVps39 might act at an earlier stage in the endo–lysosomal pathway than hVps41, as part of an intermediate CORVET/HOPS complex. Our data also show that the LAMP carrier pathway is not the only TGN exit for LAMPs. In addition to LAMP carriers, we found TGN-bound LAMP in clathrin-coated membranes [13] , [14] , which is in agreement with previous EM studies and observations showing that LAMPs can traffic directly from the TGN to early endosomes [53] . However, in contrast to CI-MPR, LAMPs were not or only moderately concentrated in clathrin-coated TGN membranes. An important implication of our findings is that the MPR and LAMP carrier pathways are independently regulated, which raises the interesting notion that subsets of lysosomal proteins could be delivered sequentially to the maturing endosomal system ( Fig. 6 ). The concentration of LAMPs in late endosomes/lysosomes is manifold higher than in early endosomes. Targeted input of LAMP proteins to late endosomes would significantly increase protein levels, as well as bypass sorting pathways active in early endosomes, for example, to intraluminal vesicles. The importance of LAMP targeting is further illustrated by the increasing number of cellular functions that requires proper LAMP levels in endo–lysosomes: sensitization to lysosomal cell death [54] ; lysosomal exocytosis [3] , cancer cell death [54] , phagosome and autophagosome maturation and fusion [3] . In addition to LAMPs, the ‘LAMP-carrier’ pathway might also be used by additional cargoes/substrates. For example, in Drosophila, Vps41/Lt was also required for the lysosomal delivery of cholesterol transporter Niemann-Pick C1 protein and the V-ATPase [29] . Targeted input of these proteins would allow a gradual assembly of a functional lysosome, for example, by preventing premature acidification and degradation. Antibodies and reagents All reagents were purchased from Sigma (St Louis, USA) unless otherwise indicated. The following antibodies were used. Mouse anti-human LAMP-1 CD107a (BD Pharmingen, San Diego, USA), rabbit anti-human LAMP-1-931.1 (M. Fukuda), rabbit anti-rat LGP120 (kind gift from I. Mellman, Genentech Inc., South San Francisco, CA, USA), mouse anti-human LAMP-2 CD107b (BD Pharmingen), rabbit anti-human LAMP-2-932.1 (M. Fukuda, Biotinylated goat anti-GFP and rabbit anti-biotin (Rockland, Gilbertsville, USA), rabbit anti-human CI-MPR GVII.16 (kind gift from S. Höning, University Cologne, Germany), rabbit anti-human ASGPR-K1 (kind gift from A. Schwartz, Washington University, St Louis, USA), rabbit anti-human albumin (Nordic, Tilburg, The Netherlands), sheep anti-human TGN46 AHP 500 (Serotec, Oxford, UK), mouse anti-bovine AP-1 100/3 (Sigma), mouse anti-HA 16B12 (Covance Research Products, New Jersey, NJ, USA) and sheep anti-rat TGN38 AHP499G f (Serotec). As bridging antibodies between mouse or sheep antibodies and protein A-gold we used rabbit anti-mouse IgG Z0412 (Dako, Heverlee, Belgium) or rabbit anti-sheep IgG H&L (Nordic, Tilburg, the Netherlands). To label endocytic compartments, we used 10 000 MW dextran-Alexa Fluor 568 or dextran-FITC (both Invitrogen) for fluorescent microscopy and 5 nm gold particles coupled to bovine serum albumin (BSA-gold 5 ) (Cell Microscopy Centre, UMC Utrecht, the Netherlands) for EM. For fluorescence, cells were grown on glass coverslips and incubated with dextran for 2 h in 1% serum containing culture medium, washed and transferred to imaging medium as described below. For immunoEM, cells were incubated with BSA-gold 5 for 2, 3 or 24 h in 1% serum containing culture medium, washed in culture medium and fixed as described below. To test lysosomal degradation of endocytosed cargo or activation of cathepsin B, cells were incubated for 4 h with DQ-BSA (Invitrogen) [55] or 2 h with Magicred cathepsin B substrate (Molecular probes) [56] , respectively, in 1% serum containing culture medium. After incubation, cells were transferred into Hanks buffered DMEM without phenol red, supplemented by 2.5% foetal bovine serum for live-cell imaging. Cell culture HepG2 cells (ATCC, clone HB-8065) were grown on 100 mm petri dishes in MEM Hanks (Invitrogen) supplemented with 10% foetal bovine serum (Sigma), 2 mM l -glutamine (Invitrogen) and 100 units per 100 μg ml −1 penicillin/streptomycin (Invitrogen) at 37 °C/5% CO 2 . HeLa cells (ATCC, clone ccl-2) were grown in DMEM (Invitrogen) supplemented with 10% foetal bovine serum, 2 mM L -glutamine and 100 units ml −1 penicillin/streptomycin at 37 °C/5% CO 2 . Transfection and immunofluorescence Human LAMP-1-mGFP (kind gift of E. Dell’Angelica [57] ) was transfected into HepG2 or HeLa cells using Effectene (Qiagen). To study LAMP trafficking, cells were grown on glass coverslips, transfected and after 16 h incubated for 2 h with dextran-Alexa568. Subsequently, cells were transferred to a Deltavision RT fluorescence microscope (Applied Precision, Issaquah, WA) and imaged in MEM Hanks without phenol red, supplemented by 2.5% foetal bovine serum, using an EMCCD camera. Cells were kept at 37 °C using a climate chamber. Images and movies were deconvolved using SoftWoRx software (Applied Precision). In an alternative protocol, cells were incubated for 1 h with dextran-Alexa568 at 5 h after transfection, then placed in a 20-°C water bath to induce a TGN block [25] , [58] , transferred to the Deltavision microscope and imaged at 37 °C 15 min after transfer. After imaging, cells were fixed in 4% wt vol −1 paraformaldehyde (PFA, Polysciences Inc.), permeabilized in 0.1% Triton X-100, labelled and embedded in Prolong gold, or Prolong DAPI (both Invitrogen). Fluorescent z-stacks were made on the Deltavision microscope (Exposure 100 ms per 300 ms, 667 frames, 200 s) and processed using SoftWoRx software. Fluorescent images were analysed using Volocity software (Volocity software Inc., Mountain View, CA, USA). siRNAs and DNA constructs In liver cells, hVps41 is expressed in two isoforms [59] , one of which contains a C-terminal RING-H2 motif possibly involved in hVps41 membrane association [59] . The RING-H2 motif containing hVps41-HA construct was cloned from hVps41 cDNA (Origene) into a pDonor201 vector (Invitrogen) using PCR. Next, a recombination reaction was performed using the Gateway system (Invitrogen) and destination vector pcDNA3dest-HA (Invitrogen) and expressed in HeLa cells. VAMP7-HA DNA, (kind gift from A. Peden, Cambridge Institute for medical research, UK), was used in a retroviral transfection system to stably transfect HeLa cells. Transfected cells were selected using geneticin and cells were grown from single colonies to yield a stable cell line. hVps41 knockdown was obtained with the on-target Smartpool human Vps41 siRNAs (no. 5: ugacauagcagcacgcaaauu, no. 6: cagcauguguauuugcauauu, no. 7: gaacggucuuggaugaacauu, no. 8: agucauaguucaagcaguuuu) (Dharmacon) using Hiperfect transfection reagent (Qiagen). hVps39 knockdown was obtained with on-target Smartpool human hVps39 siRNAs (no. 9: gcacaaaagaaacgguuca, no. 10: gcacgacgcuuucgagcca, no. 11: gugaggagguguuacggau, no. 12: ggaauacagugcuaguuga). VAMP7 knockdown was obtained using on-target smartpool siRNAs (no. 1: ggagaaagauuggaauuau, no. 2: guacucacauggcaauuau, no. 3: aagaagagguuccagacua, no. 4: gcuaagauaccuucugaaa). VPS18 knockdown was obtained using siGenome smartpool human hVPS18 siRNAs (no. 1 caaaugacccaaccacgu, no. 2 ggacaugaaccgcuucgau, no. 3 gagcuacuuugaggagauu, no. 4 gacguaaggaugacgcaaa). The knockdown phenotype for hVps41 was confirmed using the separate siRNAs from the Smartpool mix. Control cells were transfected with Allstars negative control siRNAs (indicated as scrambled control) (Qiagen). Knockdown of hVps41, hVps39, VAMP7 or hVPS18 mRNA was confirmed by RT–PCR. mRNA was isolated from cells using a RNeasy kit (Qiagen) and converted to cDNA using Tagman reverse transcriptase reagents (Applied Biosystems). Real-time PCR was performed using PCR mastermix with SYBR green (Applied Biosystems) with primers were ordered from realtimeprimers.com. Experiments were performed after 3 days silencing, which for all constructs resulted on average in 90% knockdown. Quantitative immunoEM HepG2 or HeLa cells were grown and transfected as described above. Cells were fixed by adding freshly prepared 4% w/v PFA (Polysciences) in 0.1 M phosphate buffer (pH 7.4) to an equal volume of culture medium for 5 min, followed by post-fixation in 4% w/v PFA at 4 °C overnight. Male Sprague–Dawley rats were fasted overnight and killed by CO 2 narcosis. Islets were isolated as described [60] and fixed in 4% w/v PFA. Ultrathin cryosectioning and immunogold labelling were performed as previously described [19] . In case of double-labellings, the order in which the antibodies were used is indicated on the pictures. The labelling densities of LAMP-1, LAMP-2 and CI-MPR in the TGN of HepG2 cells ( Table 1 ) were obtained from cells triple-labelled for LAMP-1 or -2, TGN46 and CI-MPR. First, labelling conditions were optimized resulting in the following order of antibodies: TGN46 (5 nm gold) × LAMP-1 or LAMP-2 (10 nm gold) × CI-MPR (15 nm gold). The triple-labellings used for quantitation were performed in duplo. Of each labelling (that is, either in combination with LAMP-1 or LAMP-2), 30 TGNs sampled from two different EM grids were photographed at 30 K and printed on photo paper of 16.5 × 23 cm 2 . LAMP and CI-MPR-representing gold particles within 20 nm from a TGN membrane were categorized as associated with clathrin-coated or non-coated membranes and expressed as percentage of total gold particles. The relative membrane length of the two TGN subdomains (that is, coated versus non-coated) was assessed by placing a transparent overlay containing a square line lattice, mesh size 10 mm, over a total of 18 TGN pictures. By counting the number of intersections of the lattice lines with the respective TGN subdomains, a measure for membrane length was obtained [61] . About 11.3% of the TGN membranes was coated and 88.7% not. Labelling densities were calculated by dividing the percentage of gold particles on a given TGN subdomain by the relative membrane length of this domain. The concentration factor of LAMPs or CI-MPR in coated TGN membranes is the ratio of the labelling densities of coated over non-coated membranes. To assess the relative distribution of LAMP carriers in control HepG2 cells, 131 LAMP-1-positive carriers (derived from two EM grids) and 148 LAMP-2-positive carriers (from three different EM grids) were counted. Counting was performed in randomly selected cell profiles, by which each encountered carrier within 150 nm from an endosome was designated endosome-associated. Early and late endosomes were identified by their number of intraluminal vesicles (ILV); early endosomes contained ≤8 ILV and late endosomes >8 ILV (ref. 20 ). Quantification of LAMP or MPR carriers in hVps41, hVps39, hVps18 or VAMP7 knockdown or scrambled control HeLa cells was performed in cells incubated for 2 h with BSA-gold 5 and immunogold labelled for LAMP-1 or CI-MPR. For each condition, the number of LAMP-1 or CI-MPR-positive carriers (vesicles smaller than 200 nm and negative for the endocytic marker BSA-gold) was quantified in 40 randomly selected cell profiles derived from two different EM grids. For each knockdown a scrambled control was taken along, from the same cell batch, which was prepared and immunogold labelled in parallel with the knockdown cells, using the same standard solutions. In Fig. 5f , the numbers for the knockdown experiments represent one experiment per condition and the numbers for the scrambled controls the average from three experiments. For each knockdown at least two independent experiments were performed to confirm the consistency of the observed phenotypes. Correlative light-electron microscopy, which combines live-cell imaging and immunogold labelling of ultrathin cryosections, was performed as described [25] . Statistics Statistics were performed using SPSS Statistics software. Normal distribution of the data was analysed using an ANOVA QC plot. The variance was analysed using a Levine test. A t -test with unequal variance was used to assess the significance of LAMP carrier accumulation. Significance was related to the scrambled control sample belonging to that specific experiment. How to cite this article: Pols, M. S. et al . hVps41 and VAMP7 function in direct TGN to late endosome transport of lysosomal membrane proteins. Nat. Commun. 4:1361 doi: 10.1038/ncomms2360 (2013).